How thermally activated deformation starts in metallic glass The studies on dynamics and deformation in glassy materials are particularly challenging because of their strongly disordered atomic structure. Here, by probing the changes in the atomic displacements and stresses at saddle points of the potential energy landscape, we show that thermally activated deformation is triggered by subnano-scale rearrangements of a small number of atoms, typically less than 10 atoms. The individual triggers are invariant of the cooling history or elastic structure of the system. However, the organizations between different trigger centres can be varied and are related to the overall stability of the system. This finding allows a semi-quantitative construction of the potential energy landscape and brings a new perspective to the study of the mechanical properties of glasses. The mechanical deformation of crystalline materials is governed by structural defects [1] , [2] , [3] , [4] , which are defined as the topological deviations from lattice periodicity. However, in amorphous materials, for example, metallic glasses, the topology of atomic connectivity varies locally and it is not obvious if the defects can be uniquely defined, even though a number of defect mechanisms of deformation have been proposed, including the concept of shear transformation zones (STZ; refs 5 , 6 ). The deformation processes in glassy systems are determined by the complicated coupling between thermal activation and external loading [7] . The pure external strain-driven scenario, for example, the athermal quasistatic (AQS) limit, has been investigated [8] , [9] , whereas in the present study, we focus our scope on the triggers of thermally activated deformation (for example, in the scenario of internal friction measurement). From the potential energy landscape (PEL) perspective [10] , [11] , two distinct processes are identified in glasses [10] , [11] , [12] , [13] ; the α processes indicate the transitions between the large-scale deep ‘meta-basins’, whereas the β processes are identified as the elementary hopping between the ‘sub-basins’ confined within a ‘meta-basin’. In general the STZ transitions correspond to the β processes and cause anelastic deformation, while percolation of such transitions are associated with the α processes and lead to macroscopic plastic flow deformation [13] , [14] , [15] . Because of the correlations with many important properties (for example, glass transition, deformation, aging, diffusion and so on), the β process is known as the key in understanding metallic glasses behaviours [16] . However, the precise identification of the β process and STZ remains elusive [16] , [17] . Different experiments [18] , [19] , [20] , [21] and simulations [5] , [15] , [22] , [23] , [24] , [25] , [26] , [27] , [28] show a large variety of STZ sizes, from few atoms to several hundred. Even similar techniques led to considerably different results. For example, in nano-indentation experiments, some studies [21] show the STZ size of few hundred atoms, while others [18] , [19] , [20] show a much smaller size around 20 atoms. These remarkable ambiguities in the size and underlying mechanism of the β process are what we seek to clarify in this work. The obtained features of the β process can be further fed into constitutive model (for example, STZ theory [25] ), which would rationalize the behaviours of metallic glasses in a multi-scale modelling framework. In most of the earlier simulation studies, the STZ is characterized by comparing the atomic configurations before and after the deformation event [22] , [23] , [24] , [25] , [26] . While this approach is valid for the systems with simple topologies (for example, crystals), it can be flawed for glassy materials, in which the structural defects are not well-defined. In fact, the relaxation of an STZ in a glassy system can affect surrounding STZs (ref. 18 ) and possibly initiate an autocatalytic process [24] or even an avalanche behaviour [29] . By comparing the atomic configurations before and after the relaxation, one actually sees the total deformation process including other affected processes. In our view the key to characterize the individual STZs is to focus on the initial triggers, which are related to the saddle points of the PEL, not the energy minimum states after deformation. By focusing on the triggers, the interferences between different STZs can be avoided, and consequently, the features of isolated STZs can be more clearly observed. Recent advances in atomistic modelling [30] , [31] , [32] made it possible to explore the underlying PEL in the glassy materials systematically, and to identify the saddle points separating neighbouring PEL minima. In the present work, we employ the activation–relaxation technique (ART; refs 33 , 34 ) to study the activation processes in a metallic glass model Cu 56 Zr 44 using an embedded-atom method potential [35] . We prepared two starting systems with different stabilities, System I and II. System I represents an unstable system, and is produced by making an instant quench to 0 K from the high temperature liquid at 2,000 K. Therefore it represents the inherent structure of a liquid at 2,000 K. System II represents a relatively more stable glass, and is produced with a finite cooling rate (1 K ps −1 ) from an equilibrated low temperature liquid at 1,000 K, a little above the glass transition temperature ( T g ~700 K), to zero temperature. To probe the β relaxation processes, that is, the local structural excitations, the initial perturbations in ART are introduced to a small group of atoms with local connectivity [36] (details in Methods section). By selecting different groups and introducing random perturbations, more than 4,000 saddle point states have been identified by ART. Admittedly, no algorithm, including ART, can guarantee the complete sampling on all existing saddle points. On the other hand, previous benchmark against experiments [31] suggests that the samplings by ART are statistically robust. Therefore, we believe the studies below based on more than 4,000 states are reasonably representative of the saddle points in the system. The system volume is fixed during the simulation. No external loads (for example, stress or shear) were introduced, and the present study deals with thermal activation-induced local deformation. As mentioned above, to avoid the mixtures of different processes, the analysis below is hereby focused on the saddle point states (that is, the trigger of the β process), rather than the states after relaxation. 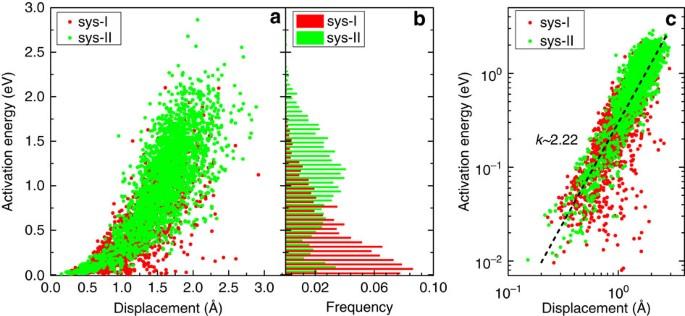Figure 1: Activation spectra and their relations with atomic displacements (a) The relation between activation energy and maximum atomic displacement on the identified saddle points. (b) The distributions of the activation energy for Systems I and II, respectively. (c) The relation between activation energy and maximum atomic displacement, on the log–log scale. Activation energy and atomic displacement Figure 1a shows the relation between the activation energy ( E act ), which is defined as the potential energy difference between the saddle point and the given initial state, and the maximum atomic displacement ( d max ) at the identified saddle point. Clearly a parabola-shaped relation can be seen, and the log-scale analysis ( Fig. 1c ) yields an exponent very close to 2. In fact, such an elastic-like behaviour is predicted by the catastrophe theory in many-body systems [37] . Figure 1b shows the distributions of the activation energies for Systems I and II. It can be seen that the unstable System I has a large fraction of low-energy excitations, whereas the relatively stable System II has more high-energy excitations. This comparison is consistent with the recent studies by Rodney et al. [7] , [30] , [38] In spite of the difference in the distribution, the data points from two systems in Fig. 1a align very well with the same parabola curve. For an elastic behaviour, the coefficient of the curve should be proportional to the shear modulus of the system. It is known that in glasses, the shear modulus mainly consist of two parts at zero temperature limit [9] , [39] , that is, the high frequency (Born) term and the non-affine term. While the non-affine term is closely related to the cooling rate history, the high frequency term is insensitive to the system’s overall stability and is almost constant for a given composition [39] . The fact that the results from the two systems yield the same parabola curve indicates that the β relaxation is affected only by the high frequency shear modulus. Such observation, in turn, is in good accordance to previous understanding that the β processes require only local rearrangements of few atoms and is insensitive to the overall properties of the system [10] , [39] . Figure 1: Activation spectra and their relations with atomic displacements ( a ) The relation between activation energy and maximum atomic displacement on the identified saddle points. ( b ) The distributions of the activation energy for Systems I and II, respectively. ( c ) The relation between activation energy and maximum atomic displacement, on the log–log scale. Full size image For elastic activation energy, the expression should be given as E act ∝ ε 2 , where ε represents the strain. The fact that in Fig. 1a indicates that there exists a constant l c , which is related to the local strain ε and the maximum atomic displacement d max , via ε ~ d max / l c . In other words, the elastic self-energy can be written as, where V eff is the effective volume for the trigger of the β relaxation and G ∞ is the high frequency shear modulus. Admittedly, if one considers an Eshelby-type inclusion scenario [5] , [40] , [41] , [42] , [43] , additional coefficient can appear in equation 1. The Eshelby factor is of the order of unity for metallic glass systems [17] , [20] , [41] , and thus in the present work we neglect this factor for simplicity. For a given interatomic potential, the high frequency atomic modulus can be readily calculated [41] , [44] . Therefore by fitting the original data in Fig. 1a to equation 1, one can obtain The result above is in a very small length scale, indicating that the β relaxation is highly localized. The specific values for V eff and l c , as well as the physical meaning of l c , will be discussed below. Atomic level stress changes and trigger atoms To further investigate the local β relaxation, we consider the atomic level stress [41] , [45] , which can describe well the local atomic environment in the metallic system [46] , [47] . In particular, the atomic level stress tensor for each atom was calculated at both the initial minimum state and identified saddle states, as and , respectively. The stress change for each atom can thus be given by . The shear component of the stress change for each atom, that is, von Mises stress, can therefore be calculated as, We then consider the relation between the changes in the atomic stress and the displacements at the saddle points. 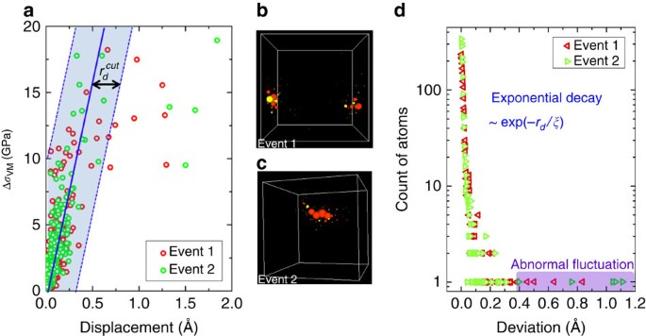Figure 2: Atomic level stresses changes and trigger atoms during deformation. (a)The relation between the atomic displacement and the stress change, for two typical excitation events. (b,c) The atomic displacements at the selected two saddle points; the radii of atoms are proportional to their displacements. Yellow particles represent Zr atoms and orange ones represent Cu atoms. (d) The distributions of deviations from the background blue line ina. Figure 2a displays such a relationship for two typical activation events. In each event, we plot the displacements and stress changes at the saddle point for every atom in the system. It can be seen that the vast majority of atoms have only small displacements and stress changes, which yield a normal fluctuation in a linear pattern (the solid blue line in Fig. 2a ). The atomic displacements at the saddle points are shown in Fig. 2b,c , where the radii of atoms are proportional to their displacements (yellow particles are Zr atoms and orange ones are Cu atoms). As seen in the figures, only few atoms have significant displacements. More importantly, the atoms with large displacements are very close to each other, which corroborate the earlier results—the trigger process of the β relaxation is highly localized. Figure 2: Atomic level stresses changes and trigger atoms during deformation. ( a) The relation between the atomic displacement and the stress change, for two typical excitation events. ( b , c ) The atomic displacements at the selected two saddle points; the radii of atoms are proportional to their displacements. Yellow particles represent Zr atoms and orange ones represent Cu atoms. ( d ) The distributions of deviations from the background blue line in a . Full size image We further calculate the statistical distance, that is, deviation, between each data point and the background fluctuation line (solid blue line in Fig. 2a ). Figure 2d shows the distribution of the deviations in a log-scale plot. It can be seen that, at small deviations, the number of atoms decreases linearly, yielding the exponential decay distribution pattern. On the other hand, there are few data points that significantly deviate from the exponential decay distribution. And the atoms with large abnormal fluctuations are related to the trigger process of the β relaxation (that is, isolated STZ). It is worth noting that, under thermal perturbations, it seems to be quite general that the responses of normal atoms (fast decay distribution) are very different from those of trigger atoms (long-tail distribution) [22] . The background exponential decay distribution can be removed by selecting appropriate cutoff distance (details in Methods section), and it is therefore possible to directly measure the number of atoms involved in a trigger process, as shown in Fig. 3 . 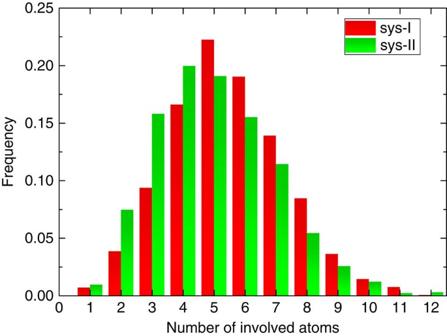Figure 3: Number of trigger atoms. The size distribution of the trigger events for the β relaxations. Red bars represent the results in System I, while green bars represent the results in System II. Figure 3: Number of trigger atoms. The size distribution of the trigger events for the β relaxations. Red bars represent the results in System I, while green bars represent the results in System II. Full size image The derived STZ sizes show a distribution with the peak position at 4–5 and maximum ~10. This demonstrates that the STZ trigger process is strongly localized and involves only a small number of atoms, which again is in excellent agreement with the analysis above. Although the macroscopic properties of System I and II are considerably different, the distributions of STZ trigger sizes are surprisingly similar to each other. Such observation raises an intriguing question: are there pre-existing defects in glasses that trigger deformation? Because it is difficult to imagine why two very different systems have the similar sizes of trigger events, if STZs are related to pre-existing defects. We should note that, through the present study we found it is difficult to predict where the triggers take place based upon the local elastic properties (for example, atomic stress and modulus). This seems in accordance to the previous study by Schuh et al. [17] , that the deformation processes in glasses are emergent and cannot be identified a priori . It is also worth stressing that the present study focuses on thermally activated deformation only. If external loading is applied, it renders the directional bias to the transition, and the system could show different deformation behaviours [7] , [30] . Under such situation, some observables (for example, low-lying modes [9] , soft spots [48] and so on) may be found to be correlated with the deformation. However, such correlations between STZs and other observables, as well as the deformation behaviours under external shear, are beyond our scope of the present work, and these subjects will be discussed separately elsewhere. We have shown above that only few atoms are involved in the triggers of β relaxation, and according to Fig. 2a , these few atoms have considerable changes in the atomic level stress at the saddle points. 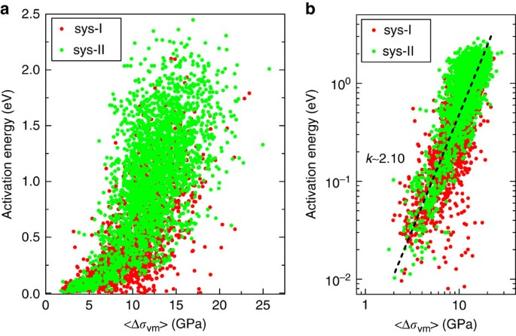Figure 4: Relations with activation energy and atomic level stress changes. (a) The relation between activation energy and maximum atomic shear stress change on the identified saddle points. (b) Plot ofaon the log–log scale. Figure 4a below shows the relation between the activation energy and the change in the average atomic level shear stress for these few atoms (note as<Δ σ VM >), for both Systems I and II. Figure 4: Relations with activation energy and atomic level stress changes. ( a ) The relation between activation energy and maximum atomic shear stress change on the identified saddle points. ( b ) Plot of a on the log–log scale. Full size image It can be seen that a parabola-shaped behaviour appears again. The log-scale plot ( Fig. 4b ) shows an overall exponent of 2.10, which indicates an elastic self-energy as, It is worth noting that the identical relation has also been discovered in studying the flow unit in metallic glass [49] . As seen in Fig. 4a the results from the two systems align with the same parabola curve, indicating the activations in two systems are affected by the high frequency shear modulus, as has been discussed earlier. By fitting the data points in Fig. 4a to equation 4, the effective volume V eff can be derived as 68.0 Å 3 . The atomic volume for Cu and Zr atoms are ~13 and 22 Å 3 , respectively, in the present modelling system. And the value of derived V eff represents a typical size of three Zr atoms or five Cu atoms, which is very well-consistent with the results in Fig. 3 . By feeding the value of V eff into equation 2, the scaling constant l c can now be resolved as 4.86 Å. The following relation between V eff and l c is then observed, Equation 5 indicates that l c is essentially the diameter of the effective volume for the trigger event, and the shape of activation unit is approximately spherical. In other words, the trigger of β relaxation is confined in a very small region with the characteristic length ~4.86 Å. During the activation, such region undergoes atomic rearrangement and yield an elastic energy increase up to the saddle point. Correlation between different triggers and PEL construction We have demonstrated above, by three different approaches, that the trigger processes of the β relaxations are strongly localized to around five atoms, and the associated activation energy can be well-described as the elastic self-energy. This result is surprisingly consistent with the X-ray experiments in metallic glasses [50] , [51] , showing that the β relaxation originates from highly localized bond switching. More importantly, the individual β processes are found insensitive to the overall properties of the system. On the other hand, however, we observe that the manner of how different β relaxation centres are organized is strongly affected by the system’s overall level of relaxation. In Fig. 5 , we show the distributions of the maximum atomic displacements at the saddle points (that is, the x -axis in Fig. 1a ) for the two systems studied. It can be seen that two systems show significantly different behaviours: the displacements are generally small in the unstable System I, whereas they are much larger in the relatively stable System II. The atomic displacements at saddle points can reflect, to some extent, the spatial separations between the neighbouring PEL minima states, and it is plausible to correlate the atomic displacements with the general coordinates of PEL (ref. 37 ). The results in Fig. 5 therefore indicate that the density of the sub-basins in the PEL is strongly related to the stability of the system. In particular, the distributions of sub-basins are very dense in an unstable system, whereas the sub-basins are rarer and more widely separated in a stable system. Such observation well-supports Stillinger’s [10] early conjecture on the distribution of the β relaxation centres. 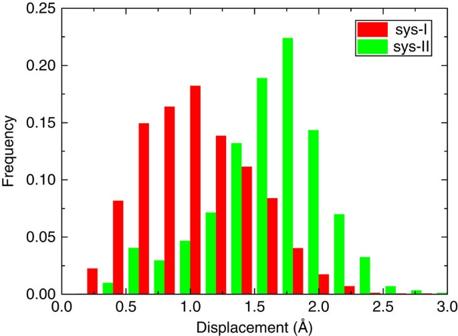Figure 5: Spatial correlation between different triggers. The distributions of the maximum atomic displacement at the saddle points. Red bars are for System I and show a smaller displacement. Green bars are for System II and yield a larger displacement. Figure 5: Spatial correlation between different triggers. The distributions of the maximum atomic displacement at the saddle points. Red bars are for System I and show a smaller displacement. Green bars are for System II and yield a larger displacement. Full size image Now, with knowing the feature of the individual β relaxation and their organization we can further construct a semi-quantitative PEL for metallic glasses as shown in Fig. 6 , adding to the previous pioneering works [13] , [14] , [52] . The meta-basin (α relaxation) has been well-investigated by Johnson et al. [13] , [14] and Maloney et al. [52] , and they show that the corresponding energy profile yields a scaling exponent of 3/2, with respect to the applied shear. The slope of meta-basin is determined by the relaxed shear modulus [39] , which is cooling rate dependent. Under a fast cooling rate, the system reaches an unstable state with a relatively low relaxed shear modulus and a shallow meta-basin. For a slow cooling rate, the system becomes more stable with a larger relaxed shear modulus and a deep meta-basin. On the other hand for β relaxations, we demonstrate that each individual sub-basin shows a history-independent elastic behaviour and is controlled by the invariant high frequency modulus G ∞ , as shown by the blue arrows in Fig. 6 . However, the organizations between different β relaxation processes can be significantly dependent on cooling history. For an unstable system, the average distances between sub-basins are quite small ; whereas for a stable system, the distributions of sub-basins are sparse and have large average separations . The larger separations of sub-basins, together with modulation by stiffer meta-basin profile, make the β activation barriers higher in a more stable system (seen in Fig.1b ). 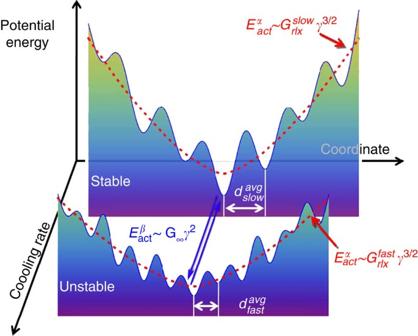Figure 6: The illustration of two-scale pattern PEL for metallic glasses. The profile of meta-basin is determined by the relaxed shear modulusGrlx=G∞+Gn.a., whereG∞is the high frequency Born term and insensitive to the cooling history,Gn.a.is the non-affine term and very sensitive to the cooling rate. A fast cooling rate leads to a smalland shallow meta-basins; a slow cooling rate leads to a largeand deep meta-basins. The individual sub-basins have similar profiles that are governed by high frequency modulusG∞, and are invariant of cooling history. However, the organizations between different sub-basins are sensitive to the overall stability of the system. The rapidly quenched system shows a small average separation, and yields smaller activation barriers, while the slowly quenched system shows a big average separation, and yields larger activation barriers. Figure 6: The illustration of two-scale pattern PEL for metallic glasses. The profile of meta-basin is determined by the relaxed shear modulus G rlx = G ∞ + G n.a. , where G ∞ is the high frequency Born term and insensitive to the cooling history, G n.a. is the non-affine term and very sensitive to the cooling rate. A fast cooling rate leads to a small and shallow meta-basins; a slow cooling rate leads to a large and deep meta-basins. The individual sub-basins have similar profiles that are governed by high frequency modulus G ∞ , and are invariant of cooling history. However, the organizations between different sub-basins are sensitive to the overall stability of the system. The rapidly quenched system shows a small average separation , and yields smaller activation barriers, while the slowly quenched system shows a big average separation , and yields larger activation barriers. Full size image We believe the constructed picture herewith can help clarify the earlier mentioned ambiguities in estimating the STZ sizes by different studies. For example, the nano-indentation experiments of Pan et al. [21] show a very large STZ size, of the order of several hundred. Their analysis is, however, based on plastic flow, which according to the picture by Johnson et al. [13] , corresponds to percolations of the meta-basins. Therefore the results are actually related to the α processes, rather than the β relaxations (that is, isolated STZs), and it is not surprising then to obtain a very large number for the estimated STZ size. In fact still with nano-indentation techniques, if one focuses on the ‘pop-in’ phenomena prior to the steady plastic flow, then a much smaller number, ~20 atoms, is obtained [18] , [19] , [20] . Because the ‘pop-in’ events are still macroscopically observable phenomena, it can therefore be inferred that 20 atoms is an upper limit of the isolated STZ size. On the other hand in atomistic simulations, Mayr [15] shows a size of 140 atoms for STZ, whereas several other studies show much smaller sizes ~10–20 (refs 22 , 23 , 24 , 25 , 26 ). In the study by Mayr [15] , the simulations are conducted under high external stress, and focused on large plastic deformation at a very short molecular dynamic timescale. Therefore the results are again more likely related to the percolations of the meta-basins, and it is reasonable to have the similar size as in the experiments by Pan et al. [21] While other studies show a much smaller size at 10–20 atoms [22] , [23] , [24] , [25] , [26] , the numbers are still obtained by comparing the initial and final (after relaxation) configurations. In our present study, however, we demonstrate that the trigger processes (that is, the saddle points) of isolated STZs involve much less than 10 atoms. It can be expected that, after relaxation, the trigger will cause other surrounding STZs or even cascade events, and more atoms would be affected. Therefore, we believe that our results are very well-consistent with the previous simulations [22] , [23] , [24] , [25] , [26] and nano-indentation experiments mentioned above [18] , [19] , [20] . To summarize, through the present study, we gain new insights on the nature of the atomic process of thermally activated deformation in metallic glasses and how they are organized in systems with different cooling rates. In particular, we found that the trigger processes of deformation consist of rearrangements of a small number (around five) of atoms with an elastic self-energy at the saddle point constituting the energy barrier, and are independent of the system’s overall properties. However, the organizations between different deformation processes can be considerably different and are closely related to the overall stability of the system. For a rapidly quenched unstable system, the spatial separations between different triggers are small and yield relatively small activation barriers, whereas for a slowly quenched stable system, the distributions of the triggers are sparse and yield higher activation barriers. Admittedly, new questions have been raised by the present study. For instance, what is the underlying mechanism for this cooling rate-dependent organization? How the correlations between different triggers (that is, isolated STZs) would further affect the deformation behaviour of the system? These challenges will warrant further studies. As a final note, the present studies on deformation mechanisms in metallic glasses enable a more comprehensive understanding to fundamental glassy physics including deformation mechanism, diffusion, glass transition, crystallization and stability of glasses and so on [16] . The obtained new insights from atomic level can be further fed into constitutive models (for example, STZ theory [25] ), which would enable the understanding and prediction to metallic glasses in a multi-scale modelling framework. In addition, based on the derived semi-quantitative PEL, we also see a considerable potential for facilitating the design of functional materials with desirable mechanical properties [53] . System set-up and details of the ART simulation We consider a metallic model system Cu 56 Zr 44 containing 2,000 atoms, interacting with an embedded-atom method potential [35] . The dimensions of the system are 32.43 × 32.43 × 32.43 Å, and periodic boundary conditions are applied to all three directions. All the simulations are under the fixed volume condition. To explore the underlying PEL, including the minima and surrounding saddle points, we employ ART, which was initially proposed by Barkema et al. [33] and further improved by Cances et al. [34] . The prepared two systems serve as the initial configurations in ART. To study the local excitations of the system, the initial perturbations in ART are introduced to a small group of atoms with local connectivity [36] . Specifically, we select an atom as the central atom, then randomly displace this atom and its first nearest neighbours, defined by the cutoff between the first and second peaks in the PDF. The magnitude of displacement is fixed at 0.5 Å, while the direction is randomly chosen. When the curvature of PEL is found to be <−0.01 eV Å −2 , the system is relaxed to the saddle point using the Lanczos algorithm [34] . The saddle point convergence criterion is fulfilled when the overall force of the total system is <0.05 eV Å −1 . The corresponding activation energy is thus the difference between the saddle point energy and the initial state energy. For each group of atoms, we employ 10 ART searches with different random perturbation directions. Since there are 2,000 such groups in our modelling system, and that overall provides 20,000 searches by ART. After removing the failed searches and redundant saddle points, 2,200 different activations, on an average, are identified for each of the prepared two systems. Removing the background exponential decay distribution The normal fluctuations, as mentioned in the main text, yield the exponential decay distribution , where the decay length ξ is actually the s.d. of the distribution. The number of atoms involved in a STZ can thus be counted by removing the atoms within normal background fluctuation. In other words, one needs to select an appropriate cutoff distance and count the number of atoms beyond this range, as illustrated in Fig. 2a . In the system with 2,000 atoms in the present study, to remove the background exponential decay distribution completely, it requires a in such a way that Otherwise, if one selects a smaller cutoff distance, even the normal fluctuation can make at least one out of 2,000 atoms located beyond , which would lead to an overestimation of the number of atoms involved in the STZ. The condition in equation 6 yields a criterion of . A systematic procedure in measuring STZ size can therefore be constructed: (i) For an identified saddle point, fit the background fluctuation line, similar to the solid blue line in Fig. 2a . (ii) Calculate the distance from each data point to the background line, and simultaneously obtain the s.d. ξ . (iii) Count the number of data points with the distance >7.6 ξ . We did the procedure to all identified saddle points, and obtained the STZ size shown in Fig. 3 . How to cite this article: Fan, Y. et al. How thermally activated deformation starts in metallic glass. Nat. Commun. 5:5083 doi: 10.1038/ncomms6083 (2014).